Elucidating electrochemical nitrate and nitrite reduction over atomically-dispersed transition metal sites Electrocatalytic reduction of waste nitrates (NO 3 − ) enables the synthesis of ammonia (NH 3 ) in a carbon neutral and decentralized manner. Atomically dispersed metal-nitrogen-carbon (M-N-C) catalysts demonstrate a high catalytic activity and uniquely favor mono-nitrogen products. However, the reaction fundamentals remain largely underexplored. Herein, we report a set of 14; 3 d -, 4 d -, 5 d - and f -block M-N-C catalysts. The selectivity and activity of NO 3 − reduction to NH 3 in neutral media, with a specific focus on deciphering the role of the NO 2 − intermediate in the reaction cascade, reveals strong correlations (R=0.9) between the NO 2 − reduction activity and NO 3 − reduction selectivity for NH 3 . Moreover, theoretical computations reveal the associative/dissociative adsorption pathways for NO 2 − evolution, over the normal M-N 4 sites and their oxo-form (O-M-N 4 ) for oxyphilic metals. This work provides a platform for designing multi-element NO 3 RR cascades with single-atom sites or their hybridization with extended catalytic surfaces. Recently, significant effort has been focused to decarbonize the production of chemicals and fuels [1] , [2] . Among these, the decarbonization of ammonia (NH 3 ) synthesis from the traditionally energy intensive and environmentally damaging Haber-Bosch (H-B) process remains a grand challenge [3] , [4] . The electrochemical synthesis of NH 3 , can ideally utilize renewable energy, reactive N-species and protons from water to generate NH 3 . The reduction of di-nitrogen (N 2 ) in aqueous protic electrolytes remains the most heavily researched green pathway for NH 3 synthesis [5] . However, due to the high bond dissociation energy of N 2 (945 kJ mol −1 ), ultra-low solubility in aqueous electrolytes and competition from the hydrogen evolution reaction (HER), the current Faradaic efficiencies (FE) and NH 3 yield rates (Yield NH3 ) remain prohibitively low [4] , [6] . Given the total lack of reproducibility and the difficulties of ubiquitous NH 3 contamination in electrochemical systems, direct N 2 reduction remains unproven in aqueous protic electrolytes [7] . To circumvent the challenges of N 2 reduction, there is a renewed interest in closing the N-cycle by recycling the reactive, more oxidized N-species (nitrate-NO 3 , nitrite-NO 2 and nitric oxide-NO) to NH 3 [8] , [9] , [10] , [11] . The electrochemical NO 3 − reduction reaction (NO 3 RR) is of particular interest due to its weaker N=O bond (204 kJ mol −1 ), large solubility in aqueous electrolytes and widespread availability. NO 3 − is an environmental pollutant found in industrial waste streams and agricultural runoffs, due to the heavy overfertilization practices currently utilized [8] . While the NO 3 RR to NH 3 provides a pathway for efficient recycling of NH 3 /NO 3 − (originating from the H-B process), additional efforts are focusing on low energy plasma techniques to produce NO 3 − from air, but such processes are to date, not energy efficient [12] , [13] , [14] . The electrochemical NO 3 RR to NH 3 is a complex 8e − (9H + ) transfer process, involving several desorbable and non-desorbable surface intermediates, creating a challenge for tailoring the catalytic surface for favorable adsorption of specific intermediates due to scaling relations [15] , [16] , [17] . Previous attempts were made to tune the intermediate adsorption binding energies by modulating the electronic structure on extended metal surfaces through alloys such as CuNi, PdAu, and PtRu [18] , [19] , [20] . These attempts achieved improved FE NH3 and Yield NH3 compared to mono-metallic counterparts, however, these approaches are still constrained by scaling relations and combat this by utilizing strongly alkaline or acidic environments with large concentrations of NO 3 − . In the biological NO 3 RR, the reaction is partitioned as an enzymatic cascade, where the initial 2e − reduction of NO 3 − -to-NO 2 − is catalyzed over a Mo-cofactor in nitrate-reductase and the further reduction of NO 2 − to NH 3 /N 2 is catalyzed over an Fe- or Cu-cofactor in nitrite-reductase [21] , [22] , [23] . Inspired by the enzymatic pathway, recent work demonstrated that an atomically dispersed bi-metallic FeMo-N-C catalyst could successfully partition the NO 3 RR into the NO 3 − -to-NO 2 − and NO 2 − -to-NH 3 constituents, outperforming its mono-metallic Mo-N-C or Fe-N-C counterparts. The atomically dispersed Mo-N x sites facilitated dissociative adsorption of NO 3 − , releasing NO 2 − , which is subsequently re-adsorbed and reduced to NH 3 over Fe-N x sites at 100% FE [24] . Additionally, other approaches to partition the NO 3 RR are emerging in the field for example, employing heterogenous metal sites, where each metal is tailored to efficiently catalyze a segment of the reaction. A recent study demonstrated potential dependent phase transitions of a Cu-Co (3–5 nm) binary metal sulfide catalyst, in which the inner Cu/CuO x phases efficiently reduce NO 3 − -to-NO 2 − , while the outer Co/CoO phases selectively reduce the NO 2 − -to-NH 3 . The latter results in a NO 3 RR cascade to NH 3 , reaching a high FE of 90.6% [25] . A recent complementary work examining a series extended of transition metal surfaces by Carvalho et al. described NO 3 RR catalyst design parameters by linking the electronic structure to experimentally observed NO 3 RR performance [26] . These design parameters are derived from microkinetic models that described the 2e − transfer rate limiting step (NO 3 − -to-NO 2 − ) and further the NO 3 RR FE NH3 , identifying a competitive adsorption between H + and NO 3 − , that was described by the material-dependent property \(({\Delta {{{{{\rm{G}}}}}}}_{{{{{{{\rm{H}}}}}}}^{*}}-{\Delta {{{{{\rm{G}}}}}}}_{{{{{{{\rm{NO}}}}}}}_{3}^{-*}})\) . The study found that increasing FE NH3 correlates with NO* binding and subsequent dissociation into N* and O* as the d-band energy approaches the Fermi energy, resulting in the Co-foil showing the highest ammonium selectivity. Atomically dispersed metal-nitrogen-carbon (M-N-C) catalysts have been extensively studied in neighboring electrocatalytic reactions (carbon dioxide reduction-CO 2 RR [27] , [28] , [29] , oxygen reduction-ORR [30] , [31] ), demonstrating excellent catalytic activities and unique reaction pathways. Recently, atomically dispersed Fe-N-C catalysts were shown to be very selective for the NO 3 RR to NH 3 [32] , [33] , owing to their maximized atomic utilization and favorable NO 3 − adsorption over H + . Additionally, isolated active sites provide an unfavorable environment for coupling adsorbed N-molecules, enabling mono N-based products (e.g., NH 3 ) to be selectively produced. The current understanding of atomically dispersed M-N-C catalysts for the complex NO 3 RR is very limited, with only M = Fe, Mo, and Cu being explored at varying conditions. Herein, we identify key transition metals and rare earth elements, important for electrocatalytic reactions and synthesize a set of 13 atomically dispersed M-N-C catalysts (M = Cr, Mn, Fe, Co, Ni, Cu, Mo, Ru, Rh, Pd, W, La, and Ce). The reaction onset potential (HER, NO 3 RR and NO 2 RR), the NO 3 RR selectivity to both NO 2 − and NH 3 and the NO 2 RR selectivity to NH 3 , elucidate several experimental activity descriptors. Isotopically doped 15 NO 2 − in the NO 3 RR highlights the complex production/consumption mechanism of the NO 2 − intermediate. Density functional theory (DFT) evaluates the Gibbs free energy for both the NO 3 RR and NO 2 RR following either the dissociative adsorption or associative adsorption pathway. Relating the experimentally determined and computationally determined activity descriptors, reveals strong correlations for the NO 2 RR ( R = 0.72) and the NO 3 RR ( R = 0.73) selectivity to NH 3 . This work bridges the gap between computation and experiment for the NO 3 − and NO 2 − reduction reactions over atomically dispersed M-N-C catalysts by providing a powerful set of activity descriptors that correlate strongly with the experimentally observed activity. These descriptors can be utilized to guide future atomically dispersed M-N x catalyst development, for highly active and efficient NO 3 − reduction to NH 3 . Structural environment of single-atom metal centers Atomically dispersed M-N-C catalysts were synthesized through the well-established sacrificial support method (SSM) originally developed by our group [34] , [35] , [36] . The SSM has been extensively applied for atomically dispersed Fe-N-C catalysts for the ORR and CO 2 RR [27] , [37] . Here, extending beyond Fe-N-C to a variety of 3 d- , 4 d- , 5 d- and f- block metals, a set of atomically dispersed M-N-C catalysts (M = Cr, Mn, Fe, Co, Ni, Cu, Mo, Ru, Rh, Pd, La, Ce, and W) were synthesized, as shown in Fig. 1a . The metallic centers ideally have a first coordination shell of 4-nitrogen atoms and are coordinated in either an in-plane or out-of-plane configuration as shown in Fig. 1b . With the synthesis conditions being adjusted to maintain the atomically dispersed nature for each metal element (Table S1 ), the resulting catalysts showed consistent porosity and pore size distribution (Fig. S1 ), degree of graphitization (Fig. S2 ) and a well-maintained metal loading at 0.5–1.5 wt% (Fig. S3 ). Fig. 1: Physical structure of the atomically dispersed transition-metal catalysts. a Selection of 3 d , 4 d , 5 d and f metals synthesized via the sacrificial support method. b Schematic of the nitrogen coordinated metal active site (M-N 4 ) on a prototype carbon matrix, illustrating in-plane and out-of-plane configurations. Where the black, blue, brown/purple balls represent carbon, nitrogen and metal atoms, respectively. c – e Representative atomic resolution HAADF STEM images for the Fe-N-C, Rh-N-C and La-N-C catalysts. High contrast points indicate atomically dispersed metal sites. Corresponding EDS mapping of the M-N-C is given below. Full size image X-ray diffraction (XRD) shows only the characteristic (002) and (100) peaks for carbon, confirming the absence of bulk-like ordered metallic phases (Fig. S4 ). 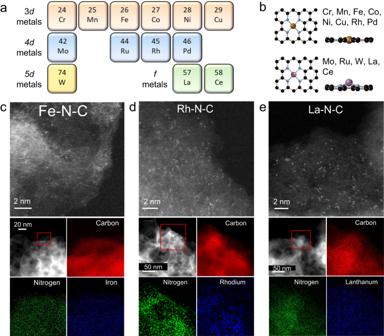Fig. 1: Physical structure of the atomically dispersed transition-metal catalysts. aSelection of 3d, 4d, 5dandfmetals synthesized via the sacrificial support method.bSchematic of the nitrogen coordinated metal active site (M-N4) on a prototype carbon matrix, illustrating in-plane and out-of-plane configurations. Where the black, blue, brown/purple balls represent carbon, nitrogen and metal atoms, respectively.c–eRepresentative atomic resolution HAADF STEM images for the Fe-N-C, Rh-N-C and La-N-C catalysts. High contrast points indicate atomically dispersed metal sites. Corresponding EDS mapping of the M-N-C is given below. Figure 1c–e shows representative aberration corrected high-angle annular dark-field scanning transmission electron microscopy (AC-HAADF-STEM) images for the Fe, Rh, and La-N-C, where atomically dispersed metal sites are clearly observed through the high contrast points. Energy dispersive X-ray spectroscopy (EDS) maps confirm the homogenous distribution of carbon, nitrogen, and the relevant metal throughout the catalyst, Fig. 1c–e (see other M-N-Cs in Figs. S5 – S8 ). Throughout the main text physical characterization of the Fe-, Rh- and La-N-C are shown as a 3 d , 4 d and f -metal representative for the set of M-N-C catalysts. Complete characterization for the remaining M-N-Cs is found in the ESI as noted. The electron energy loss spectroscopy (EELS) in Fig. 2a–c shows the EELS spectra of small sample regions containing single atoms of Fe, Rh, and La, respectively. The EELS point spectra show the co-existence of the N K-edge and the corresponding metal-edge (Fe-L 3,2 , Rh-M 3 , La-M 5 , 4 ), supporting the bond formation between the singe metal atom and supporting nitrogen atoms (M-N x ). X-ray absorption spectroscopy (XAS) was used to further investigate the chemical state and coordination environment of the catalysts, including X-ray absorption near-edge structure (XANES) and extended X-ray absorption fine structure (EXAFS). The XANES edge position and features (e.g., the intensity of the while line) of the Fe K-edge (7112 eV), Rh K-edge (23,219.9 eV) and La L 3 -edge (5890.6 eV) as compared to their corresponding reference foil and oxide compounds indicate oxidation states of ca . Fe 2+ , Rh 3+ , and La 3+ , in agreement with the Fe 2 p , Rh 3 d and La 3 d X-ray photoelectron spectroscopy (XPS) analysis (Fig. 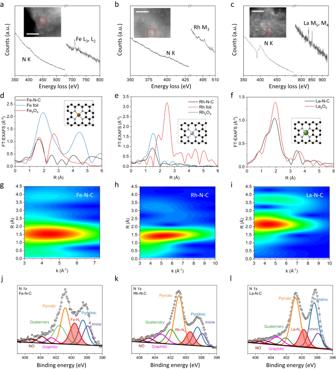Fig. 2: Coordination environment of the single-atom metal centers. a–cAtomic resolution EELS point spectra of the N K-edge and corresponding metal-edge of Fe (L3,2), Rh (M3) and La (M5,4), in the M-N-C catalysts, indicating nitrogen coordination of the single atom M-Nxsite. All scale bars are 2 nm.d–fFT EXAFS spectra of the Fe, Rh and La-N-C catalysts, with the corresponding metallic foil and metal oxide standards, demonstrating the presence of M-Nxsites. Where the black, blue, brown/silver/green balls represent carbon, nitrogen and metal atoms, respectively.g–iWT-EXAFS of the Fe K-edge of Fe-N-C, Rh K-edge of Rh-N-C and La L3-edge of La-N-C.j–lN 1sXPS spectra for the Fe, Rh and La-N-C catalysts, confirming the presence of M-Nxmoieties. S9 ). Interestingly, for Cr-N-C, evaluated to be one of the most selective M-N x sites for the conversion of NO 3 − to NH 3 (Fig. 3d ), the XANES analysis reveals a relatively high Cr oxidation sate, comprising a mixture Cr 6+ (20–30%) and Cr 3+ (70–80%). Analogously for other M-N-C catalysts, the chemical state of the metal center is assessed by their respective XANES and XPS spectra (Figs. S10 – S16 ). Furthermore, the EELS valence state analysis for Fe-N-C and La-N-C, evaluating the intensity ratio and separation distance between the Fe L 3 /L 2 and La M 5 /M 4 edges further supports the oxidation state of Fe (between Fe 2+ and Fe 3+ ) and La (La 3+ ) (Fig. S17 ). However, the Rh K-edge EELS signal is too weak to perform quantitative analysis. EXAFS provides structural information of the metal centers inner coordination spheres, confirming the presence of shorter bonds (M-C/M-N/M-O) rather than longer metallic M-M bonds. From comparison with complementary techniques (EELS and XPS) the formation of M-N bonds is supported. Fourier transformed (FT) EXAFS spectra for the Fe K-edge, Rh K-edge and La L 3 -edge, respectively are shown in Fig. 2d–f . In the Fe-N-C and Rh-N-C spectra, a single sharp peak was observed at a bond distance of ca. 1.5 Å (phase uncorrected) for both, characteristic of the Fe-N and Rh-N coordination in the first shell. While for La-N-C, an f -metal with a complex coordination environment (shown to sit out of plane during the modeling of the active site, Fig. 1b ) a peak was observed at higher distances between 1 and 2.5 Å (phase uncorrected). A similar peak can also be observed in the FT-EXAFS of amorphous La 2 O 3 . Therefore, we assume that in our La-N-C sample a strongly disordered local environment around the single atom site, including the possible formation of small metal oxide-clusters. For the Ce-N-C catalyst, a more complex peak split feature was observed indicating the complex nature of f -metal M-N-C catalysts (Fig. S18 ). To deconvolute minor contributions to the EXAFS spectra at larger bond distances, wavelet transforms of the EXAFS oscillations, providing high resolution information in both k-space and R-space are shown in Fig. 2g–I . For Fe-N-C, Rh-N-C, and La-N-C, in addition to the high intensity Fe-N, Rh-N and La-N peak, a low intensity peak is observed at ca . 3.5 Å, 3.2 Å, and 3.7 Å (at low k-space values), respectively which we attribute to Fe-C, Rh-C, and La-C interactions in the second coordination shell. The lack of peaks in wavelet-transformed EXAFS spectra at higher values of wavenumber k indicates the absence of metal-metal bonds in the M-N-C catalysts, and, hence, absence of metallic or large oxide clusters. FT-EXAFS and WT-EXAFS for the M-N-C and corresponding metal oxide standards are given for Fe-, Rh-, and La-N-C in Fig. S19 , while complete XANES, EXAFS, and FT-EXAFS spectra are provided for all M-N-Cs in Figs. S10 – S12 , with fitting parameters provided in Table S2 and fitting results plotted in R-space found in Fig. S20 , respectively. Fig. 2: Coordination environment of the single-atom metal centers. a – c Atomic resolution EELS point spectra of the N K-edge and corresponding metal-edge of Fe (L 3,2 ), Rh (M 3 ) and La (M 5,4 ), in the M-N-C catalysts, indicating nitrogen coordination of the single atom M-N x site. All scale bars are 2 nm. d – f FT EXAFS spectra of the Fe, Rh and La-N-C catalysts, with the corresponding metallic foil and metal oxide standards, demonstrating the presence of M-N x sites. Where the black, blue, brown/silver/green balls represent carbon, nitrogen and metal atoms, respectively. g – i WT-EXAFS of the Fe K-edge of Fe-N-C, Rh K-edge of Rh-N-C and La L 3 -edge of La-N-C. j – l N 1 s XPS spectra for the Fe, Rh and La-N-C catalysts, confirming the presence of M-N x moieties. Full size image Fig. 3: Electrochemical activation, selectivity, and activity for the NO 3 RR and NO 2 RR. a Example of a linear sweep voltammetry (LSV) curve for the Cr-N-C catalyst in electrolytes of 0.05 M PBS (HER), 0.05 M PBS + 0.01 M KNO 2 (NO 2 RR) and 0.05 M PBS + 0.16 M KNO 3 (NO 3 RR). Representative LSV over the metal free N-C and a variety of 3 d and 4 d metals for the ( b ) NO 3 RR and ( c ) NO 2 RR. Complete LSV for all examined M-N-C and metal free catalysts are given in Fig. S28 . d Gap analysis plot (GAP) for the electrochemical NO 3 RR for all M-N-C catalysts in 0.05 M PBS + 0.16 M KNO 3 for 2 h. The top section of the figure shows the Faradaic efficiency for NO 2 − (blue; top-down) and NH 3 (gray; bottom-up) as a function of the applied potentials between −0.2 V and −0.8 V vs. RHE. A horizontal line is set at 50% FE to guide the eye. The bottom section of the figure shows the corresponding yield rate (μmol h −1 cm −2 ) for NO 2 − (blue; triangle) and NH 3 (gray; circle) as a function of the applied potentials. The corresponding NO 3 RR chronoamperometry plots and UV–Vis detection for NO 2 − and NH 3 concentrations are shown in Figs. S29 – 38 . Error bars are determined from three replicate trials at −0.40 V vs. RHE. The GAP for the metal free N-C catalysts is shown in Fig. S39 . Full size image XPS was used to further examine the metal-nitrogen coordination and other nitrogen moieties present. The representative N 1s spectra for the Fe-, Rh-, and La-N-C catalysts in Fig. 2j–l , reveals the presence of metal-nitrogen moieties (M-N x ). N 1 s XPS spectra for the remaining M-N-C catalysts is shown in Figs. S21 – 24 , all of which demonstrate the formation of M-N x moieties. The deconvoluted high resolution N 1 s XPS spectra showed a variation in the N-content and N-moiety percentage (e.g., pyridinic, pyrrolic, graphitic metal-N x ), as shown in Tables S3 – 6 . In summary, 13 atomically dispersed M-N-C catalysts have been synthesized using the SSM. By combining AC-STEM, EELS, XAS and XPS, the atomically dispersed nature of each metal site has been comprehensively visualized and confirmed to be in a M-N x coordination. Critically, the well-deciphered coordination environment of the metal center allows us to elucidate the intrinsic activity of the different M-N x moieties towards the electrocatalytic transformation of reactive N-species. Electrochemical performance The NO 3 RR is somewhat universal in that even metal-free nitrogen-doped-carbon (N-C) showed limited but observable activity towards the generation of NH 3 and NO 2 − under an isotopically labeled 15 NO 3 − feed in neutral electrolyte (pH = 6.3 ± 0.05) at −0.4 (V vs. RHE) (Fig. S25 ). Comparatively, with the addition of nitrogen-coordinated metal sites Cr-N-C as an example, the FE NH3 increased from ca . 10% (metal free N-C) to 91.2 ± 9.6%. While the introduction of Fe-N x sites boosted the FE NH3 to 99.1 ± 2.6% (again at −0.4 V vs. RHE) and the corresponding Yield NH3 increased from 1.3 to 10.0 ± 1.3 μmol h −1 cm −2 . It should be noted that, for the NO 3 RR activity, as compared to measurements performed in neutral media, the current density and NH 3 yield rate could be significantly enhanced under alkaline conditions, while maintaining a high FE NH3 . Given Fe-N-C as an example, Fig. S26 shows that when using a 1 M KOH electrolyte (pH = 13.8 ± 0.17), the NH 3 partial current density increased from 2 mA cm −2 (11.4 μmol h −1 cm −2 ) to 35 mA cm −2 (156.5 μmol h −1 cm −2 ) at −0.4 V and further to 175 mA cm −2 (750.4 μmol h −1 cm −2 ) at −0.6 V, both with a FE NH3 above 95%. Other work on alkaline NO 3 RR also found similar trends [18] , [33] , [38] . However, as a fundamental study, this work focused on neutral pH (pH 6.3 ± 0.05) to evaluate the intrinsic activity of the M-N x sites toward the electrocatalytic NO 3 RR and NO 2 RR. Regardless of the NO 3 RR pathways [39] , [40] , [41] , the surface intermediates *NO 2 and *NOOH are inevitable before the reaction pathway diverges to its several possible products. The NO 2 − molecule is also the first desorbable reaction intermediate, playing a key role in the NO 3 RR via a cascade pathway [24] , [42] . For the set of M-N-C catalysts in this work, the NO 2 RR displayed an earlier activation than the NO 3 RR by linear sweep voltammetry (LSV), as shown in Fig. 3a , indicating that the 6e − transfer from NO 2 − /*NOOH to NH 3 , in the NO 3 RR was more facile than the initial 2e − transfer from *NO 3 − to *NO 2 − /*NOOH, which is the rate limiting step and thus the focus of the computational work in the following discussion. Representative LSV for the metal free N-C and a variety of 3 d and 4 d metals demonstrates the range of NO 3 RR (Fig. 3b ), and NO 2 RR (Fig. 3c ) activities, with Cu-N x being the most active NO 3 RR site and Fe-N x being the most active NO 2 RR site. As a unique nitrate-to-nitrite electrocatalyst [24] , Mo-N-C was even more inert than the metal free N-C. A full analysis of the reaction onset potentials (Fig. S27 ) clearly visualizes the range of onset potentials for the diverse M-N x sites. To investigate the NO 3 RR activity and selectivity towards NH 3 and NO 2 − , a series of 2-h potential holds were performed at potentials between −0.2 V and −0.8 V. A gap analysis plot (GAP) was constructed in Fig. 3d to visualize the nitrogen conversion landscape. Collectively, as the cathodic potential decreased, the yield rate of NH 3 and NO 2 − increased for all catalysts, but the selectivity varied. Specifically, both Fe-N-C and Cr-N-C showed the highest NH 3 selectivity (FE NH3 92–100%) at −0.4 V and −0.6 V. In contrast, Mo-N-C showed comparable, consistent, and somewhat potential-independent selectivity for NO 2 − (40–50% FE NO2- ) and NH 3 (50–55% FE NH3 ), as expected given that Mo-N x sites were shown in our previous work, as an active nitrate-to-nitrite converter via dissociative adsorption (chemical process) [24] . Similarly, the Mn-, Pd-, W-, La-, and Ce-N-C showed moderate NO 2 − and NH 3 selectivity at high overpotentials (~70% FE NH3 vs. ~30% FE NO2- ) and the FE for nitrogen conversion (FE NH3 + FE NO2- ) was maintained at 100%. Other early transition metals (Co-, Ni- and Cu-N-C) showed irregular potential dependence on selectivity, wherein Co-N-C showed a volcano trend for FE NH3 but consistent FE NO2- and the nitrogen conversion was far below 100% FE through the entire potential range. For an easier comparison, the NO 3 RR electrolysis results (FE NH3/NO2- and Yield NH3/NO2- ) have been separated based on the applied potential in Fig. S40 , where its clearly observed that Cr-N-C was leading the other catalysts between −0.2 V and −0.6 V, being exceptional at −0.2 V (9.33 μmol h −1 cm −2 and 94% FE NH3 ). However, Ni-N-C and Cu-N-C showed a strong potential dependence on the Yield NH3 , where Cu-N-C rivals Cr-N-C at −0.8 V (61 vs. 59 μmol h −1 cm −2 ). Particularly, Cu-N-C maintained 100% FE for NH 3 + NO 2 − (FE NH3 = 72%) at −0.8 V, indicating that no current is wasted on the parasitic HER. Two distinct exceptions were Ru-N-C and Rh-N-C, albeit their early activation indicated by LSV (Fig. 3 ), both of which showed inferior NH 3 and NO 2 − activity (Fig. 3d ), displaying unique and significant gaps between the NH 3 and NO 2 − FE bars. This gap in FE is likely due to insoluble, undetected gas phase products (Fig. S41 ), likely from the HER, as the isolated active sites present in atomically dispersed catalysts are unfavorable for the coupling of N-N bonds for N 2 . It was recently observed for the NO 3 RR and previously reported for the CO 2 RR that under a cathodic potential, atomically dispersed Cu-N x sites can reduce to form metallic clusters and even nanoparticles at more cathodic potentials [43] , [44] , [45] . Interestingly, additional investigations employing operando XAS over other atomically dispersed transition metal sites (M = Mn, Fe, Co, Ni and Pd) revealed a stable atomically dispersed M-N x site, even under highly reductive potentials [46] , [47] , [48] , [49] . 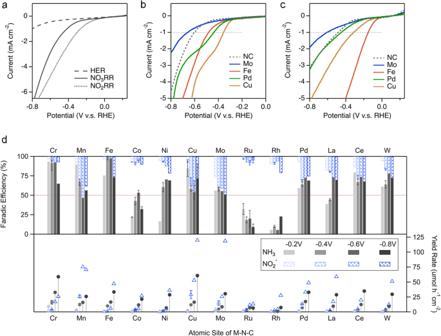Fig. 3: Electrochemical activation, selectivity, and activity for the NO3RR and NO2RR. aExample of a linear sweep voltammetry (LSV) curve for the Cr-N-C catalyst in electrolytes of 0.05 M PBS (HER), 0.05 M PBS + 0.01 M KNO2(NO2RR) and 0.05 M PBS + 0.16 M KNO3(NO3RR). Representative LSV over the metal free N-C and a variety of 3dand 4dmetals for the (b) NO3RR and (c) NO2RR. Complete LSV for all examined M-N-C and metal free catalysts are given in Fig.S28.dGap analysis plot (GAP) for the electrochemical NO3RR for all M-N-C catalysts in 0.05 M PBS + 0.16 M KNO3for 2 h. The top section of the figure shows the Faradaic efficiency for NO2−(blue; top-down) and NH3(gray; bottom-up) as a function of the applied potentials between −0.2 V and −0.8 V vs. RHE. A horizontal line is set at 50% FE to guide the eye. The bottom section of the figure shows the corresponding yield rate (μmol h−1cm−2) for NO2−(blue; triangle) and NH3(gray; circle) as a function of the applied potentials. The corresponding NO3RR chronoamperometry plots and UV–Vis detection for NO2−and NH3concentrations are shown in Figs.S29–38. Error bars are determined from three replicate trials at −0.40 V vs. RHE. The GAP for the metal free N-C catalysts is shown in Fig.S39. Further studies employing post-mortem STEM observed atomically dispersed sites after reductive potentials in the CO 2 and N 2 reduction reactions, over Ru-, Rh-, Ce-N-C, and other rare earth metals [50] , [51] , [52] , [53] , [54] . To investigate possible morphological changes to the atomically dispersed nature of the catalysts in this work after the NO 3 RR electrolysis, the representative Fe-, Rh-, and La-N-C catalysts were imaged. Post-mortem STEM images in Figs. S42 – S44 confirm atomically dispersed nature of the Fe-, Rh- and La-N x sites after the series of NO 3 RR electrolysis from −0.2 to −0.8 V for 2 h each. It is important to note that post-mortem STEM does not reveal possible in-situ restructuring under electrolysis conditions. However, as reported in a recent study employing Cu-N-C for the NO 3 RR, as morphological reconstructions were occurring as a result of the cathodic potential, a significant increase in the current is readily observed over time in the electrochemical response (chronoamperometry curves) as the Cu-N x sites transformed into metallic Cu clusters/particles [43] . Similar changes in the electrochemical response would be expected in the current study during both the NO 3 RR and NO 2 RR if significant morphological reconstruction was occurring, however, this was not observed. This may suggest, however not confirm without operando XAS, that even for Cu-N-C (which has been shown to be more susceptible to morphological changes under reductive potentials than other M-N-C catalysts), significant morphological reconstruction of the Cu-N x sites may not be occurring. Perhaps because of variations in the stability of the Cu-N x sites, originating from the different M-N-C synthesis approaches and precursor selections. This behavior is observed in the literature for Cu-N-C, by comparing operando studies under reductive potentials, for which some studies report active site reconstruction at −0.2 V vs. RHE [43] and others report no changes up to −0.6 V vs. RHE [44] . Additionally, at the mild cathodic potential in this work of −0.2 V, at which the correlations (discussed in the following section) are most accurate, significant morphological reconstruction may not be expected and was not observed over time in the electrochemical NO 3 RR and NO 2 RR performances, however, direct spectroscopic evidence would be required to confirm this hypothesis. Although no M-N x restructuring was observed through post-mortem STEM (Fe-, Rh-, and La-N-C) or suggested by the electrochemical response, this cannot be totally ruled out and will require future operando XAS studies for a robust evaluation. For the role of potential nitrite (as a by-product or intermediate), previous reports usually considered the NO 3 RR as a direct 8e − transfer pathway with certain irreversible NO 2 − desorption or leaching [32] , [33] , [55] . Here, doping of isotopic 15 NO 2 − in the NO 3 RR, schematically shown in Fig. 4a , revealed that trace amounts (e.g., 1 ppm) of 15 NO 2 − could be easily reduced to 15 NH 3 even under a concentrated 14 NO 3 − environment (10,000 ppm), which applied to both M-N x sites and metal-free N-C sites (Figs. S45 – 46 ). 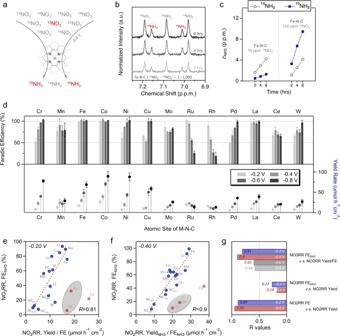Fig. 4: Mechanistic analysis of the NO3RR via a NO2−intermediate, NO2RR performance and experimental correlations between lining NO3RR selectivity and NO2RR performance. a–cIsotopic analysis of competing NO3RR and NO2RR reactions at −0.4 V.aSchematic for NO3RR electrolysis in which small amounts of15NO2−are doped in 0.16 M14NO3−.bNMR spectra for the electrolysis with 10 ppm of15NO2−doped in 0.16 M14NO3−(10,000 ppm), sampled at 2, 4, and 6 h.cTime course analysis of14NH3and15NH3concentration at 2, 4, and 6 h for the NO3RR with 10 ppm15NO2−(left) and 100 ppm15NO2−(right) in 0.16 M14NO3−(10,000 ppm).dElectrochemical NO2RR for M-N-C catalysts in 0.05 M PBS + 0.01 M KNO2for 0.5 h. Faradaic efficiency for NH3as a function of the applied potential between −0.2 V and −0.8 V (top). Bottom section shows the corresponding NH3yield rate. The chronoamperometry plots and UV-Vis detection curves for NH3are shown in Figs.S50–56. Note, FE’s over 100% arise from electrolyte dilution to bring the concentration of NH3into the UV-vis calibrated range. Error bars are determined from three replicate trials. Correlations between the NO3RR Faradaic efficiency for NH3in Fig.3d, whereRis the correlation coefficient (y-axis) and the dividend of the NH3yield rate and Faradaic efficiency of the NO2RR in Fig. 4d at (e) −0.20 V and (f) −0.40 V. The NO2RR, YieldNH3/FENH3is represented as the NO2RR total current (NO2RR, jtotal). The correlation between the NO2RR, YieldNH3and NO3RR, FENH3is shown in Fig.S57. Ru and Rh outliers (gray shades) were excluded from the linear fit due to the dominant NO3RR gaseous products as shown in Fig.S41as well as Co-N-C.gSummary of the correlation coefficients,R, for varying experimental NO3RR-NO2RR correlations. Correlations not shown in Fig. 4e, f, are shown graphically in Figs.S58–60. Figure 4b shows the NMR spectra for a time course electrolysis over Fe-N-C, wherein even at a concentration ratio of 1,000:1 ( 14 NO 3 − : 15 NO 2 − ), the 15 NO 2 − competed for an active site, yielding comparable 15 NH 3 . NMR spectra for the other M-N-C catalysts is shown in Fig. S47 , where a similar trend is observed for most metals with the no exception of Co- and Ni-N-C, where significantly more isotopic 15 NH 3 is generated than standard 14 NH 3 , in support of Fig. 3d , suggesting their poor activity towards NO 3 − but high activity towards NO 2 − , which will be addressed in the following section. As the concentration ratio is reduced to 100:1 ( 14 NO 3 − : 15 NO 2 − ), the 15 NO 2 − outcompeted 14 NO 3 − , yielding significantly more 15 NH 3 than 14 NH 3 over the 6-h electrolysis (Fig. 4c ). This indicates that for the nitrogenous products in the NO 3 RR, the potential participation of bulk NO 2 − or locally channeled NO 2 − , significantly complicates the mechanism of NH 3 production (e.g., 2e − + 6e − vs. 8e − ) [24] , [56] . Therefore, unambiguously identifying whether the underlying reaction mechanism is a direct 8e − pathway, a (rapid) 2e − + 6e − pathway with a bulk/channeled NO 2 − intermediate, or a combination thereof, is of great significance for the design and optimization of NO 3 RR systems and even more complex nitrate-involving reactions [57] , [58] . Fig. 4: Mechanistic analysis of the NO 3 RR via a NO 2 − intermediate, NO 2 RR performance and experimental correlations between lining NO 3 RR selectivity and NO 2 RR performance. a – c Isotopic analysis of competing NO 3 RR and NO 2 RR reactions at −0.4 V. a Schematic for NO 3 RR electrolysis in which small amounts of 15 NO 2 − are doped in 0.16 M 14 NO 3 − . b NMR spectra for the electrolysis with 10 ppm of 15 NO 2 − doped in 0.16 M 14 NO 3 − (10,000 ppm), sampled at 2, 4, and 6 h. c Time course analysis of 14 NH 3 and 15 NH 3 concentration at 2, 4, and 6 h for the NO 3 RR with 10 ppm 15 NO 2 − (left) and 100 ppm 15 NO 2 − (right) in 0.16 M 14 NO 3 − (10,000 ppm). d Electrochemical NO 2 RR for M-N-C catalysts in 0.05 M PBS + 0.01 M KNO 2 for 0.5 h. Faradaic efficiency for NH 3 as a function of the applied potential between −0.2 V and −0.8 V (top). Bottom section shows the corresponding NH 3 yield rate. The chronoamperometry plots and UV-Vis detection curves for NH 3 are shown in Figs. S50 – 56 . Note, FE’s over 100% arise from electrolyte dilution to bring the concentration of NH 3 into the UV-vis calibrated range. Error bars are determined from three replicate trials. Correlations between the NO 3 RR Faradaic efficiency for NH 3 in Fig. 3d , where R is the correlation coefficient (y-axis) and the dividend of the NH 3 yield rate and Faradaic efficiency of the NO 2 RR in Fig. 4d at ( e ) −0.20 V and ( f ) −0.40 V. The NO 2 RR, Yield NH3 /FE NH3 is represented as the NO 2 RR total current (NO 2 RR, j total ). The correlation between the NO 2 RR, Yield NH3 and NO 3 RR, FE NH3 is shown in Fig. S57 . Ru and Rh outliers (gray shades) were excluded from the linear fit due to the dominant NO 3 RR gaseous products as shown in Fig. S41 as well as Co-N-C. g Summary of the correlation coefficients, R , for varying experimental NO 3 RR-NO 2 RR correlations. Correlations not shown in Fig. 4e, f, are shown graphically in Figs. S58 – 60 . Full size image Figure 4d (and shown individually by applied potential in Figs. S48 – 49 ) shows the NO 2 RR electrolysis for all M-N-C catalyst under a 0.01 M NO 2 − feed, a concentration mimicking the bulk NO 2 − concentrations in the NO 3 RR electrolysis (Fig. 3d ). Obviously, both the NH 3 selectivity and activity of the NO 2 RR were significantly higher than that of the NO 3 RR (Fig. 3d ) for all catalysts. Specifically, Fe-, Co-, and La-N-C showed 100% FE NH3 over the whole potential range and Cr-, Ni-, Cu-, Pd-, and W-N-C showed increasing FE NH3 as the cathodic potentials decreased, reaching 100% at −0.8 V. Again, Mo-N-C showed a unique and potential-independent FE NH3 around 75%. Similar to the NO 3 RR, the NO 2 RR for Ru-N-C and Rh-N-C showed a distinct decreasing trend on the FE NH3 and consistent Yield NH3 over the entire potential range, likely being outcompeted by the HER as the cathodic potential decreased. To examine the relationship between the NO 2 RR and NO 3 RR, Fig. 4e, f correlates the activity of NO 2 RR (Yield NH3 /FE NH3 ) with the selectivity of NO 3 RR (FE NH3 ), revealing a linear relationship at −0.20 V and −0.40 V. This linear relationship suggests a major contribution from the bulk or locally channeled NO 2 − towards NH 3 (2e − + 6e − pathway). Meanwhile, the correlation between the FE NO2- in the NO 3 RR and the Yield NH3 in the NO 2 RR, has a poor linear fit (Fig. S59 ), highlighting the complex reaction mechanism. In contrast, the poor correlations between the NO 3 RR FE NO2- and NO 2 RR Yield NH3 (Fig. 4g ), confirmed that in the NO 3 RR the bulk NO 2 − species were in a complex production-consumption process rather than an irreversibly desorbed final by-product. Computational descriptors for the NO 3 RR and NO 2 RR As discussed above, the first 2e − transfer is the rate limiting step in the NO 3 RR, therefore DFT was used to study the energetics of key intermediates in the conversion of NO 3 − -to-NO 2 − on various catalytic active sites (Fig. S61 ). This included the *NO 3 surface intermediate formed by oxidative associative adsorption of NO 3 − , the *O surface intermediate formed by neutral dissociative adsorption of NO 3 − [24] , and the *NO 2 surface species formed in the reductive adsorption of NO 3 − , these result in four thermodynamic reaction descriptors, as shown in Fig. 5a . Fig. 5: Computational NO 3 RR descriptors as calculated by using DFT with optB86b-vdW functional. a Gibbs free energies (∆ r G) of the reaction for the first two electron transfer steps in the NO 3 RR. Processes that generate NO 2 − in the bulk electrolyte are shown in blue. Note solid bars indicate no electron transfer, uphill gradient stripes indicate a reductive e − transfer and downhill gradient stripes indicate an oxidative/reverse electron transfer. b Quadrant plot of the ∆ r G for associative adsorption \([{\,\! }^{*}+{{{{{{\rm{NO}}}}}}}_{3}^{-}\to {\,\! }^{*}{{{{{{\rm{NO}}}}}}}_{2}]\) (Y 1 -axis), dissociative adsorption \([{\,\! }^{*}+{{{{{{\rm{NO}}}}}}}_{3}^{-}\to {\,\! }^{*}{{{{{{\rm{O}}}}}}+{{{{{\rm{NO}}}}}}}_{2}^{-}]\) (X-axis) and *NO 2 desorption \([{\,\! }^{*}{{{{{{\rm{NO}}}}}}}_{2}\to {\,\! }^{*}+{{{{{{\rm{NO}}}}}}}_{2}^{-}]\) (Y 2 -axis), forming sectors where certain reaction pathways are thermodynamically favored. The main quadrants were determined by the X-axis and Y 1 -axis. Quadrants III and IV were further divided by the Y 2 -axis into III.a, III.b, IV.a and IV.b sub − sections. The three reaction coordinates determined two types of NO 3 − adsorptions and two types of NO 2 − evolutions as shown by the diagram above the figure. For simplified plots correlating two descriptors at a time, see Fig. S63 . c Correlation between DFT-derived \({\Delta }_{{{{{{\rm{r}}}}}}}{{{{{\rm{G}}}}}}[{\,\! }^{*}+{{{{{{\rm{NO}}}}}}}_{3}^{-}\to {\,\! }^{*}{{{{{{\rm{NO}}}}}}}_{2}]\) and experiment-derived NO 3 RR FE NH3 at −0.2 V vs. RHE. d Correlation between DFT-derived \({\Delta }_{{{{{{\rm{r}}}}}}}{{{{{\rm{G}}}}}}[{\,\! }^{*}+{{{{{{\rm{NO}}}}}}}_{2}^{-}\to {\,\! }^{*}{{{{{{\rm{NO}}}}}}}_{2}]\) and experiment-derived NO 2 RR FE NH3 at −0.2 V vs. RHE. Oxygenated active sites (O-M) were included for the oxyphilic elements (Mo, La, Ce and W), where R is reported as the absolute value of the correlation coefficient. 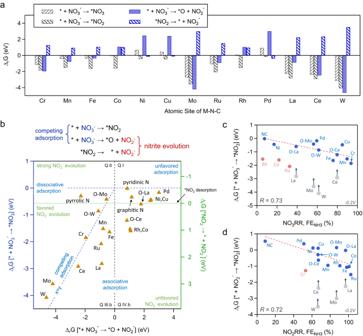Fig. 5: Computational NO3RR descriptors as calculated by using DFT with optB86b-vdW functional. aGibbs free energies (∆rG) of the reaction for the first two electron transfer steps in the NO3RR. Processes that generate NO2−in the bulk electrolyte are shown in blue. Note solid bars indicate no electron transfer, uphill gradient stripes indicate a reductive e−transfer and downhill gradient stripes indicate an oxidative/reverse electron transfer.bQuadrant plot of the ∆rG for associative adsorption\([{\,\!}^{*}+{{{{{{\rm{NO}}}}}}}_{3}^{-}\to {\,\!}^{*}{{{{{{\rm{NO}}}}}}}_{2}]\)(Y1-axis), dissociative adsorption\([{\,\!}^{*}+{{{{{{\rm{NO}}}}}}}_{3}^{-}\to {\,\!}^{*}{{{{{{\rm{O}}}}}}+{{{{{\rm{NO}}}}}}}_{2}^{-}]\)(X-axis) and *NO2desorption\([{\,\!}^{*}{{{{{{\rm{NO}}}}}}}_{2}\to {\,\!}^{*}+{{{{{{\rm{NO}}}}}}}_{2}^{-}]\)(Y2-axis), forming sectors where certain reaction pathways are thermodynamically favored. The main quadrants were determined by the X-axis and Y1-axis. Quadrants III and IV were further divided by the Y2-axis into III.a, III.b, IV.a and IV.b sub−sections. The three reaction coordinates determined two types of NO3−adsorptions and two types of NO2−evolutions as shown by the diagram above the figure. For simplified plots correlating two descriptors at a time, see Fig.S63.cCorrelation between DFT-derived\({\Delta }_{{{{{{\rm{r}}}}}}}{{{{{\rm{G}}}}}}[{\,\!}^{*}+{{{{{{\rm{NO}}}}}}}_{3}^{-}\to {\,\!}^{*}{{{{{{\rm{NO}}}}}}}_{2}]\)and experiment-derived NO3RR FENH3at −0.2 V vs. RHE.dCorrelation between DFT-derived\({\Delta }_{{{{{{\rm{r}}}}}}}{{{{{\rm{G}}}}}}[{\,\!}^{*}+{{{{{{\rm{NO}}}}}}}_{2}^{-}\to {\,\!}^{*}{{{{{{\rm{NO}}}}}}}_{2}]\)and experiment-derived NO2RR FENH3at −0.2 V vs. RHE. Oxygenated active sites (O-M) were included for the oxyphilic elements (Mo, La, Ce and W), whereRis reported as the absolute value of the correlation coefficient. Full size image Figure 5a shows that the Mo-N 4 , La-N 4 , Ce-N 4 , and W-N 4 sites could strongly adsorb NO 3 − ( ∆ r G ~ −4eV) in a dissociative manner, forming an *O surface species and a free NO 2 − molecule. For these oxyphilic metals, upon exposure to NO 3 − molecules, the single-atom sites are oxygenated with a fifth ligand and the new active site (O-M-N 4 ) can still coordinate a NO 3 − /NO 2 − molecule for further reduction [24] . Figure S62 shows that the O-M-N 4 sites had a weaker interaction with NO 3 − but could stabilize the *NO 3 /*NO 2 surface intermediates. For the Cr-N 4 , Mn-N 4 , Fe-N 4 , and Ru-N 4 sites, associative and dissociative adsorption of NO 3 − is likely a competitive process that also depends on the cell potential. Namely, while the associative adsorption of NO 3 − is potential dependent, dissociative adsorption is not as no electrons are involved in this process. Co-N 4 , Ni-N 4 , Cu-N 4 , Pd-N 4 , and La-N 4 sites adsorb NO 3 − associatively and produce NH 3 via a *NO 2 intermediate. Additionally, our DFT descriptors suggest limited NO 3 RR activity over Rh-N 4 sites, being only favorable via the reductive adsorption of NO 3 − , while in other computational based works, Rh-N 4 sites suffer some competition between *H and *NO 3 , in agreement with the poor NO 3 RR activity observed in our experimental observations [41] , [59] . The quadrant plot in Fig. 5b graphically shows the correlations between the DFT-derived descriptors, mapping out the competitive NO 3 − adsorption and sources for NO 2 − evolution. Specifically, the far ends of Quadrant I, Quadrant II and Quadrant IV.b represent unfavored NO 3 − adsorption, exclusive NO 2 − evolution and unfavored NO 2 − evolution, respectively. These three blank sectors explain the above-mentioned universal NO 3 RR activity for all M-N-C and metal free N-C catalysts (Fig. S64 ), as well as the variant but non-dominant FE NO2- in the NO 3 RR. The diagonal of Quadrant III ( x = y ) indicates competitive associative and dissociative adsorption of NO 3 − . The largest NO 2 − producing catalyst, Mo-N-C (O-Mo-N 4 and Mo-N 4 sites), is located at the diagonal, indicating comparable associative and dissociative adsorption. Several metal centers (e.g., Mn, Fe, Ru, La, and Ce) fall below the diagonal in Quadrant III.b and upper Quadrant IV.b, suggesting a favored associative NO 3 − adsorption for high NH 3 selectivity in NO 3 RR electrolysis (Fig. 3d ). Quadrant IV.b (Co, Rh, O-Ce and O-La) marks the region where a solely direct 8e − pathway to NH 3 is feasible, with formation of the *NO 2 intermediate being favored, while both descriptors for the generation/desorption of NO 2 − are unfavored. Quadrant IV.a (Ni, Cu and Pd, pyridinic-N and graphitic-N) shows a weak stabilization of the *NO 2 intermediate, while simultaneously showing activity for the desorption of *NO 2 for NO 2 − evolution. It should be noted that Mo-N-C is the only metal center favoring NO 2 − evolution through both the dissociative NO 3 − adsorption and *NO 2 desorption paths, explaining the unique selectivity of Mo-N-C in the NO 3 RR (Fig. 3d ). The DFT calculated Gibbs free energy changes for these descriptors are given in Table S7 . To evaluate the practical relevance of these computational descriptors, a set of correlations were developed between the DFT-derived free energies (∆ r G) in Fig. 5a and the electrocatalytic performance in Figs. 3d and 4d . Specifically, Fig. 5c shows the correlation between the adsorption energy of NO 3 − ( \({\Delta }_{{{{{{\rm{r}}}}}}}{{{{{\rm{G}}}}}}[{\,\! }^{*}+{{{{{{\rm{NO}}}}}}}_{3}^{-}\to {}^{*}{{{{{{\rm{NO}}}}}}}_{2}]\) ) and the NO 3 RR NH 3 selectivity (FE NH3 ), wherein a linear correlation ( R = 0.73) is observed at −0.2 V. This result highlights the importance of a stable *NO 2 intermediate for high NH 3 selectivity in both the 8e − pathway or the 2e − + 6e − pathway (which requires the re-adsorption of NO 2 − ). Additionally, the involvement of the oxo-form for the highly oxyphilic elements (O-Mo, O-W, O-La, O-Ce) shifts them back onto the trend line as compared to their bare M-N 4 counterparts. These results suggest the distinct active sites/reaction mechanism of early transition 4 d- , 5 d- and f- metal-based M-N-C catalysts in neutral environments, which could be attributed to the oxophilicity and large coordination number of these metals that allow simultaneous coordination of multiple intermediates [60] . Similarly, Fig. 5d shows a comparable correlation ( R = 0.72) between the adsorption energy of NO 2 − ( \({\Delta }_{{{{{{\rm{r}}}}}}}{{{{{\rm{G}}}}}}[{\,\! }^{*}+{{{{{{\rm{NO}}}}}}}_{2}^{-}\to {}^{*}{{{{{{\rm{NO}}}}}}}_{2}]\) ) and the NO 2 RR ammonia selectivity (FE NH3 ), indicating that the stabilization of the *NO 2 intermediate also plays a key role in the NO 2 RR as well as the downstream 6e − transfer in the NO 3 RR. It is important to note potential limitations of these computational-experimental correlations. From our observations, metal centers over which H* adsorption is a competing factor leading to the HER dominating (Ru- and Rh-N-C, Fig. 3 ) the NO 3 RR are not well predicted by these correlations. Similarly, metal centers which demonstrate significant NO 2 − activation, with poor NO 3 − activation (observed over Co-N-C in the isotopic NO 2 − doping experiments, Fig. S47 ) are also not well predicted by these correlations. However, the NO 3 RR FE NO2- showed minimum correlations with either \({\Delta }_{{{{{{\rm{r}}}}}}}{{{{{\rm{G}}}}}}[{\,\! }^{*}{{{{{{\rm{NO}}}}}}}_{2}\to {\,\! }^{*}+{{{{{{\rm{NO}}}}}}}_{2}^{-}]\) or \({\Delta }_{{{{{{\rm{r}}}}}}}{{{{{\rm{G}}}}}}[{\,\! }^{*}+{{{{{{\rm{NO}}}}}}}_{3}^{-}\to {\,\! }^{*}{{{{{{\rm{O}}}}}}+{{{{{\rm{NO}}}}}}}_{2}^{-}]\) , as shown in Fig. S65 . This agrees well with the above-mentioned poor correlation between the NO 3 RR FE NO2- and NO 2 RR Yield NH3 (Figs. 4g and S59 ), wherein the bulk NO 2 − species in the NO 3 RR were in an active but and complex production-consumption process, making it difficult to deconvolute the NO 2 − production and consumption rates from its net yield. In summary, a rich set of atomically dispersed 3 d -, 4 d -, 5 d -, and f -block M-N-C catalysts with a well-established M-N x coordination was synthesized. The gap analysis plot revealed diverse NO 3 RR performance, wherein Cr-N-C and Fe-N-C were the most NH 3 selective catalysts, achieving near 100% FE NH3 , while Mn-, Cu-, and Mo-N-C were highly selective for NO 2 − . For the NO 2 RR, several elements including Cr-, Fe-, Co-, Ni-, Cu- and La-N-C achieved a FE NH3 of 100% at high overpotentials, with Fe and Co-N-C showing 100% FE NH3 over the entire potential range. Isotopically doped 15 NO 2 − in concentrated 14 NO 3 − , demonstrated the ease at which minute concentrations of NO 2 − in the bulk electrolyte can preferentially reduce to NH 3 , convoluting the possibility of a direct 8e − pathway or a 2e − + 6e − cascade pathway with NO 2 − as transient intermediate for the NO 3 RR. The correlation between experimental NO 3 RR ammonia selectivity and experimental NO 2 RR activity suggested a universal contribution of the NO 2 − intermediate in NO 3 RR (2e − + 6e − ). The DFT-derived thermodynamic descriptors can theoretically explain the electrocatalytic selectivity for each metal center. Furthermore, these computational descriptors showed good correlations with the experimental performances, such that a simple computationally evaluated descriptor can be utilized to estimate the activity of M-N-C catalysts for the NO 3 RR and NO 2 RR. While these computational-experimental activity descriptors provide correlations for the NO 3 RR and NO 2 RR activity, these correlations are limited when the H + adsorption is a competing factor leading to the HER over NO 3 RR (Ru- and Rh-N-C) and when there is poor NO 3 − activation in contrast with significant NO 2 − activation (Co-N-C). Importantly, these computational-experimental activity descriptors are based on the M-N x active site and have strong predictive NO 3 /NO 2 RR ability at low potentials, where the intrinsic nature of the M-N x site is observed. However, the effectiveness of these activity descriptors decreases as the overpotential increases, forcibly driving the reaction and possibly inducing structural changes to the M-N x sites, convoluting the intrinsic activity of the atomically dispersed metal center. This work deciphered the unique fundamentals of the NO 3 RR over atomically dispersed M-N-C catalysts to create a set of experimentally driven computational descriptors for the NO 3 /NO 2 RR activity, paving the road for the design of tandem NO 3 RR systems and nitrate-containing systems composed of either multi-metallic M-N-C catalysts or extended catalytic surfaces supported by synergistic M-N-C supports. Materials Nicarbazin (Sigma-Aldrich), CAB-O-SIL® LM-150 fumed silica (Cabot), Aerosil® OX-50 (Evonik), iron(III) nitrate nonahydrate (Sigma-Aldrich), chromium(III) acetylacetonate (Sigma-Aldrich), manganese(II) nitrate tetrahydrate (Sigma-Aldrich), cobalt(II) nitrate hexahydrate (Sigma-Aldrich), nickel(II) nitrate hexahydrate (Sigma-Aldrich), copper(II) nitrate hemi pentahydrate (Sigma-Aldrich), ammonium molybdate tetrahydrate (Sigma-Aldrich), ruthenium(III) nitrosylnitrate (Alfa Aesar), rhodium(III) nitrate hydrate (Sigma-Aldrich), palladium(II) nitrate dihydrate (Sigma-Aldrich), lanthanum(III) nitrate hexahydrate (Alfa Aesar), cerium(III) nitrate hexahydrate (Fisher Scientific) and ammonium paratungstate (Sigma-Aldrich), potassium nitrate (Sigma-Aldrich), potassium nitrite (Sigma-Aldrich), isotopic potassium nitrate ( 15 N, 99% - Cambridge Isotope Laboratories), isotopic sodium nitrite ( 15 N, 98% + - Cambridge Isotope Laboratories). Synthesis of atomically dispersed M-N-C catalysts All catalysts were synthesized following the well-established sacrificial support method, as detailed below, with the metal precursor loading, pyrolysis temperature, pyrolysis atmosphere and etching environment being tuned to maintain atomically dispersed metal sites between the different metals (Supplementary note 1 ). Synthesis of Mn, Fe, Co, Ni, Cu, Mo and W-N-C catalysts First a slurry of a carbon-nitrogen containing precursor, Nicarbazin (6.25 g), the silica sacrificial support, LM-150 (Cabot, 1.25 g), OX-50 (Evonik, 1.25 g) and Stöber spheres (made in house, 0.5 g) and the corresponding metal salt precursor (Mn = 0.266 g, Fe = 0.60 g, Co = 0.272 g, Ni = 0.271 g, Cu = 0.345 g, Mo = 0.262 g and W = 0.095 g), in 50 mL of MilliQ water was created. Next, the slurry was sonicated for 30 min before being dried overnight at 45 °C, under constant stirring. The mixture was then further dried in an oven at 45 °C for 24 h. The resulting powder was then ball milled at 45 Hz for 1 h. The catalyst powder is then pyrolyzed at 975 °C (with a ramp rate of 15 °C min −1 ) under a reductive H 2 /Ar (7%/93%) atmosphere for 45 min. The pyrolyzed powder is then ball milled a second time at 45 Hz for 1 h. The silicate template is then etched in a hydrofluoric acid (15 M) solution for 96 h. The catalyst is then recovered by filtration and washed to neutral pH, followed by drying at 60 °C overnight. The catalyst undergoes a second pyrolysis in a reductive NH 3 /N 2 (10%/90%) atmosphere at 950 °C for 30 min (with a ramp rate of 20 °C min −1 ). The catalyst is then ball milled a final time at 45 Hz for 1 h. Synthesis of Cr-N-C catalyst The synthesis is identical to the previous procedure, with only the pyrolysis temperatures being reduced to 650 °C in both the first and second pyrolysis, to maintain an atomic dispersion of the Cr metal. The metal salt precursor loading of Cr = 0.519 g. Synthesis of Ru-N-C catalyst The synthesis is identical to the previous procedure, with the pyrolysis temperatures being reduced to 650 °C and an inert argon pyrolysis atmosphere, to maintain an atomic dispersion of the Ru metal. The metal salt precursor loading of Ru = 0.235 g. Synthesis of Rh and Pd-N-C catalysts The synthesis is identical to the previous procedure, with the high pyrolysis temperatures of 975 °C and 950 °C for the first and second pyrolysis, respectively, however the pyrolysis is performed in an inert argon atmosphere, to maintain an atomic dispersion of the Rh and Pd metals. The metal salt precursor loading of Rh = 0.215 g and for Pd = 0.198 g. Synthesis of the La and Ce-N-C catalysts The synthesis is identical to the previous procedure, with the pyrolysis temperatures being reduced to 650 °C under an inert argon pyrolysis atmosphere. Furthermore, the etching of the silica template was performed in an alkaline 4 M NaOH environment at 80 °C for 96 h. If etched using a hydrofluoric acid environment, the La and Ce readily form LaF 3 and CeF 3 nanoparticles. The metal salt precursor loading of La = 0.060 g and Ce = 0.061 g. Physical characterization The physical structure and atomically dispersed nature of the catalysts were analyzed by aberration-corrected scanning transmission electron microscopy (AC-STEM) and EDS using a JEOL ARM300CF at an accelerating voltage of 300 kV. The coordination environment and valence state of the atomically dispersed sites were examined through atomic resolution electron energy loss spectroscopy (EELS) on a Nion UltraSTEM200 microscope equipped with a cold FEG, a C3/C5 aberration correction and a high-energy resolution monochromated EELS system (HERMES). To mitigate the beam damage on the coordination between single metal atoms and nitrogen-carbon support, the EELS was collected at a low voltage of 60 kV. During acquisition, the energy dispersion was set as 0.16 ~ 0.3 eV/channel with an exposure time of 2–4 s nm −2 . The background in each spectrum was removed by a power-law function and the de-noising of the spectra was performed by the multivariate weighted principal component analysis routine in the Digital Micrograph software. The hierarchical pore structure of the catalyst was examined by scanning electron microscopy (SEM) on an FEI Magellan 400 XHR SEM. The electronic structure and local bonding environment of the metal sites were analyzed by ex-situ X-ray Absorption Spectroscopy (XAS) collected on several beamlines. Rh K-edge was measured on the SAMBA beamline at SOLEIL synchrotron radiation facility, Paris, France. The sample was measured in fluorescence mode and references in transmission mode using a Si (220) monochromator for the energy selection. Ionization chambers to measure the X-ray intensity before and after the sample were filled with a mixture of Ar/N 2 ( I 0 ) or pure Ar ( I 1 / I 2 ). The La L 3 -edge was measured on the XAFS beamline at ELETTRA synchrotron radiation facility, Triest, Italy. The sample was measured in transmission mode using a Si (111) 20% detuned monochromator for the energy selection. Simultaneously, a vanadium reference foil was measured for the energy calibration. Ionization chambers to measure the X-ray intensity before and after the sample were filled with a mixture of N 2 /He ( I 0, I 1 , I 2 ). The Fe K-edge was measured on the lab-based easyXAFS300 at the Fritz Haber Institute, Berlin, Germany (measured in transmission mode). Using a Ge (620) crystal for the energy selection and a Si drift detector (AXAS-M assembly from KETEK GmbH). A W-ProtoXRD X-ray tube was used. The Ce L 3 -edge, Cr, Mn, Co, Ni and Cu K-edge were measured on the KMC-3 beamline at the Bessy synchrotron radiation facility, Berlin, Germany. Cr-N-C in transmission mode, Cu-, Co-, Ni-, Mn- and Ce-N-C in fluorescence mode using a Si (111) monochromator for the energy selection. The ionization chamber for the measurement of the X-ray intensity before the sample was filled with 100 mbar air ( I 0 ). Either a 13 element Si drift detector was used (fluorescence) or PIPS detector (transmission). Note that the energy resolution of the XAS spectra measured at the KMC-3 beamline is compromised due to technical issues involving the optics/mirrors at the KMC-3 beamline. However, the samples and corresponding reference foils and compounds were measured for energy calibration and comparison of features. Note Mo-N-C and Pd-N-C were measured on the 10-BM beamline of the Advanced Photon Source at Argonne National Laboratory. The ATHENA software was used for data alignment and XAS spectra extraction [61] . A set of in-house built Wolfram Mathematica scripts were used for the XANES analysis. Fitting of the EXAFS spectra was done using FEFFIT scripts [61] . The photoelectron amplitudes and phases were calculated by the FEFF8 code [62] . The EXAFS R-space fitting parameters and results are given in Table S8 . If the M-N-C sample and corresponding reference material were not measured at the same beamline (Cr-, La-, and Ce-N-C) the S 0 2 factor multiplied by the coordination number is reported. The metal valence state and quantification of nitrogen-moieties of the M-N-C catalysts were analyzed by XPS. The XPS was performed on a Kratos AXIS Supra spectrometer with a monochromatic Al Kα source (with an emission current of 15 mA and X-ray power of 225 W, while for the high-resolution spectra the emission current and power are 20 mA and 300 W, respectively). No charge neutralization was employed as all these samples are highly conductive, carbon-based catalysts. Survey spectra were obtained at a pass energy of 160 eV from 1400 eV to 5 eV at a step size of 1 eV. The High-resolution C 1s, N 1s and O 1s spectra were obtained at a pass energy of 20 eV with a 0.1 eV step size. The metal spectra were obtained at a pass energy of 40 eV with a 0.1 eV step size. A C 1s spectra was also obtained at a pass energy of 40 eV for calibration. CasaXPS software was used to analyze and fit all spectra and all spectra were calibrated based on the sp 2 carbon (284 eV). A Linear background was employed for the C 1s and N 1s spectra, while a Shirley background was used for the O 1s and metal spectra. The sp 2 carbon in the C 1s spectra was fit with a 80% Gaussian/20% Lorentzian function and all other spectra were fit using a 70% Gaussian/30% Lorentzian function. All fitting parameters employed in this work are based on previous fittings from our group that are reported in the literature references here for this class of M-N-C catalysts [63] , [64] , [65] , [66] . X-ray diffraction (XRD) patterns were collected on a Rigaku Ultima-III powder X-ray diffractometer. Inductively coupled plasma mass spectrometry (ICP-MS) on an Aligent 5110 was performed to accurately quantify the low metal content of the M-N-C catalysts. N 2 physisorption was recorded on a Micromeritics 3Flex Analyzer at 77 K, using a low-pressure dosing mode (5 cm 3 g −1 ). The surface area and pore size distribution were obtained using the Brunauer–Emmett–Teller method and the non-local density functional theory model (NLDFT), respectively. Raman spectra were obtained with a 633 nm laser and 600 g.mm grating, using a Horiba LabRAM-HR. Preparation of the working electrode% A catalyst ink was created by mixing 10 mg of catalyst in a solution of 680 μL IPA, 300 μL MilliQ water and 20 μL of a 5 wt% Nafion solution and sonicated for 1 h. For linear sweep voltammetry (LSV) experiments, 12.35 μL of catalyst ink was drop cast on a glassy carbon electrode (0.247 cm 2 ) for a catalyst loading of 0.5 mg cm −2 . For chronoamperometry experiments an AvCarb MGL370 carbon paper was used as the working electrode. The carbon paper was pre-treated by plasma cleaning for 15 min to remove the PTFE layer and then subsequently washed in 3 M H 2 SO 4 and MilliQ water to create a hydrophilic surface. After the pretreatment, 12.5 μL of catalyst ink was drop cast on the carbon paper with a 0.25 cm 2 geometric working area for a catalyst loading of 0.5 mg cm −2 . Linear sweep voltammetry Note that the applied potential for all electrochemical tests is not iR corrected. From PEIS measurements (from 1 MHz to 1 Hz at 7 points per decade), the solution and contact resistances are small at 13.5 Ω, aided by the high concentration of KNO 3 , which dissociates into K + and NO 3 − ions, creating a strong electrolyte with a high conductivity. To evaluate the onset potentials for the HER, NO 2 RR, and NO 3 RR, LSV was performed. All LSV measurements were obtained on a Biologic potentiostat, using a rotating disk electrode in a single compartment cell. A glassy carbon electrode (0.247 cm 2 ), graphite rod and reversible hydrogen electrode are used as the working, counter, and reference electrodes, respectively. To evaluate the HER onset potential, a 0.05 M PBS electrolyte was used. For the NO 2 RR onset potential LSV was performed in a 0.05 M PBS + 0.01 M KNO 2 electrolyte. For the NO 3 RR onset potential LSV was performed in a 0.05 M PBS + 0.16 M KNO 3 electrolyte. LSV curves were obtained by sweeping reductively from 1 V to −1 V vs. RHE at 5 mV s −1 at a rotation speed of 1600 rpm. The reaction onset potential was determined to be the potential at which a current density of 0.4 mA cm −2 was reached. Electrocatalytic nitrate reduction Electrochemical nitrate reduction measurements were carried out in a customized two compartment H-cell, as shown in Fig. S66 separated by a Celgard 3401 porous polypropylene membrane (used without pre-treatment). Electrochemical measurements were recorded using an AutoLab potentiostat. A standard three-electrode system was used with a reversible hydrogen electrode (HydroFlex®) and a graphite rod as the reference and counter electrode, respectively. The electrolyte used for all nitrate reduction experiments is a 0.05 M phosphate buffer solution (PBS) and with 0.16 M NO 3 − (KNO 3 ). The electrolyte pH was measured to be pH = 6.3 ± 0.05 using an Orion Dual Star pH probe. Error bars are obtained from measurements on three independent electrolytes. Prior to electrochemical tests, N 2 gas (research grade 99.9995% - PraxAir) is purged in both the working and counter chambers for 30 min at 80 sccm, which contain 30 mL and 25 mL of electrolyte, respectively. To assess if saturating the electrolyte with N 2 or Ar has an impact on the equilibrium potentials of the NO 3 RR processes, open circuit voltage measurements were performed under N 2 or Ar saturation and showed negligible differences as shown in Fig. S67 . Potentiostatic tests are performed for 2 h under constant stirring at a constant N 2 gas flow rate of 20 sccm to the working chamber. Potentiostatic tests were performed at potentials of −0.20, −0.40, −0.60 and −0.80 V vs. RHE. After the electrolysis, the electrolyte in both the working and counter chambers was sampled and tested for NH 3 and NO 2 − . Note that at the pH = 6.3 ± 0.05 conditions utilized in this work, the pKa of ammonia has not been reached (pKa 9.2), therefore the ammonia produced is in the protonated form ammonium (NH 4 + ). However, in the alkaline conditions present during the Berthelot method for detection, the NH 3 /NH 4 + is present in the NH 3 form. Therefore, the discussion in this manuscript is for the detected product ammonia (NH 3 ). Note our previous work has demonstrated that these atomically dispersed M-N-C catalysts have been shown to be inactive for the reduction of N 2 under these conditions [24] . NO 3 RR tests in alkaline media (pH = 13.8 ± 0.17) were performed using a 1 M KOH + 0.16 M KNO 3 electrolyte. Due to the extremely high NH 3 yield rate, potentiostatic tests were performed for 15 min at potentials of −0.20, −0.40, −0.60, and −0.80 V vs. RHE. Electrocatalytic nitrite reduction Electrochemical nitrite reduction experiments were performed analogously to nitrate reduction experiments. The electrolyte is 0.05 M PBS and 0.01 M NO 2 − (KNO 2 ) (pH = 6.26 ± 0.11). Due to the higher NH 3 yield rates of the more active NO 2 RR, potentiostatic tests were performed for 30 min. Potentiostatic tests were performed at potentials of −0.20, −0.40, −0.60, and −0.80 V vs. RHE. After each electrolysis, the electrolyte in the working chamber was sampled and tested for NH 3 detection. Isotope-labeling experiments Isotopic nitrate 15 NO 3 − labeling Isotopic 15 NO 3 − labeling experiments were performed by using K 15 NO 3 (99% - Cambridge Isotopes) as the isotopic nitrate source with a 0.05 M PBS + 0.16 M K 15 NO 3 − electrolyte (pH 6.3 ± 0.05). Isotopic 15 NO 3 − experiments were performed using a metal free N-C catalyst. Using a metal free N-C catalyst simultaneously allows the source of the N in the produced NH 3 to be confirmed, while also demonstrating that the even the metal free N-moieties in the N-C catalysts can catalyze the NO 3 RR (and is not from N-originating from catalyst decomposition).Electrolysis was performed at −0.40 V for 4 h, after which the electrolyte in the working chamber was samples and the produced 15 NH 3 was quantified by 1 H NMR. Isotopic nitrite 15 NO 2 − labeling Isotopic 15 NO 2 − labeling experiments were performed by using Na 15 NO 3 (98% + - Cambridge Isotopes) as the isotopic nitrite source. Isotopically labeled 15 NO 2 − at concentrations of 100, 10, and 1 ppm were doped into the 0.05 M PBS + 0.16 M KNO 3 (10,000 ppm NO 3 − ) electrolyte. Potentiostatic tests were performed at −0.40 V vs. RHE for 6 h, under constant stirring and a N 2 gas flow of 20 sccm to the working chamber. The electrolyte was sampled at 2-, 4-, and 6-h time intervals and the 15 NH 3 was quantified by 1 H NMR. Calculation of the yield and faradaic efficiency Note that all error bars in this work are determined from triplicate experiments on independently prepared electrodes and are then calculated using a 90% confidence interval. For the nitrate (NO 3 − ) and nitrite (NO 2 − ) reduction reactions, the NH 3 yield rate was calculated by Eq. ( 1 ). Yield_NH_3=c_NH_3 * V/Mw_NH_3 * t * A_electrode
 (1) For the nitrate (NO 3 − ) and nitrite (NO 2 − ) reduction reactions, the NH 3 Faradaic efficiency was calculated by Eq. ( 2 ). FE_NH_3=n * F * c_NH_3 * V/Mw_NH_3 * Q
 (2) In the NO 3 RR, the nitrate (NO 3 − ) to nitrite (NO 2 − ) reduction Faradaic efficiency was calculated by Eq. ( 3 ). FE_NO_2^-=n * F * c_NO_2^- * V/Mw_NO_2^- * Q
 (3) where \({{{{{{\rm{c}}}}}}}_{{{{{{{\rm{NH}}}}}}}_{3}}\) is the concentration of NH 3(aq) (μg mL −1 ), V is the volume of the electrolyte (mL), \({{{{{{\rm{Mw}}}}}}}_{{{{{{{\rm{NH}}}}}}}_{3}}\) is the molar mass of NH 3 (17.031 g mol −1 ), t is the duration of the chronoamperometric measurement (h), the surface area of the working electrode, A electrode is 0.45 cm 2 . The number of electrons transferred, n , for NO 3 − to NO 2 − is n = 2 and for NO 3 − to NH 3 is n = 8. F is Faraday’s constant (96,485 C mol −1 ), the concentration of NO 2 − (μg mL −1 ), C NO2- , where the molar mass of NO 2 − , Mw NO2- is (46.005 g mol −1 ) and the charge during the chronoamperometric measurement, Q. Product detection For typical, non-isotopically labeled NO 3 RR and NO 2 RR electrolysis, products were quantified using an ultraviolet-visible (UV–Vis) spectrophotometer (Shimadzu, UV−2600). Determination of ammonia Ammonia was quantified by UV–Vis using the Berthelot reaction. In cases producing large concentrations of NH 3 , the working electrolyte solution was diluted such that the absorbance would fall within the range of the calibration curve. Specifically, 2 mL of the electrolyte (or diluted electrolyte if needed) was pipetted into a vial. To this, 2 mL of a 1 M NaOH solution that contains 5 wt% salicylic acid, and 5 wt% sodium citrate was added. Next, 1 mL of a 0.05 M NaClO and 0.2 mL of a 1 wt% C 5 FeN 6 Na 2 O (sodium nitroferricyanide) was added to the solution. The solution was incubated in the dark at ambient condition for 1 h, then UV-Vis spectra were recorded. The concentration of NH 3 is determined using the maximum absorbance at a 655 nm wavelength, when compared to the generated calibration curves, Figs. S68 – 69 . Determination of nitrite Nitrite was quantified by UV–Vis using a commercial NO 2 − assay kit (Spectroquant), based on the Griess test. In cases producing large concentrations of NO 2 − , the working electrolyte solution was diluted such that the absorbance would fall within the range of the calibration curve. Specifically, 2 mL of the electrolyte (or diluted electrolyte if needed) was placed in a vial. To this, 22 mg of the assay reagent was added to the electrolyte and incubated in the dark at ambient conditions for 10 min. After incubation, the UV–Vis spectra were taken, and the concentration of nitrite was determined at a maximum absorbance of 540 nm wavelength, when compared to the generated calibration curves, Fig. S70 . NMR determination of ammonia For isotopic labeling experiments, nuclear magnetic resonance (NMR) spectroscopy was used to detect and quantify both 14 NH 3 and 15 NH 3 . Dimethylsulfoxide-d6 (DMSO) and 3-(trimethylsilyl)-1-propanesulfonic acid sodium salt (DSS) were used as the locking solvent and internal standard, respectively. For the NMR test solution, 580 μL of the electrolysis electrolyte, 25 μL of DMSO, 20 μL of 3 M H 2 SO 4 , and 75 μL of 6 mM DSS (made with Millipore water) are mixed. The NMR spectrum was obtained on a Bruker CRYO 500 MHz spectrometer. The signal from H 2 O was restrained for better accuracy by applying the solvent suppression method during acquisition. Topspin 4.0.8 software was used to process the NMR data. Standard NMR calibration curves for standard 14 NH 3 and isotopically labeled 15 NH 3 are shown in Fig. S71 . Computational details All the DFT calculations were performed with the generalized gradient approximation approach and projector augmented-wave pseudopotentials [67] , [68] using the Vienna Ab initio Simulation Package [69] , [70] , [71] . To account for the van der Waals interactions, an optB86b-vdW functional was used [72] , [73] , [74] , [75] with a gamma centered 8 × 8 × 1 (M-N 4 sites, pyridinic N, graphitic N) or 3 × 3 × 1 k -mesh (pyrrolic NH) and Fermi-smearing. Sigma and the plane-wave basis cutoff was set to 0.03 and 400 eV, respectively. We approached modeling of the M-N 4 sites in the M-N-C catalysts by creating two carbon atom vacancies in the graphene, in which we place a metal atom [27] , [65] , [76] , [77] , [78] . Structures were then optimized as neutral, using unrestricted open shell spin density and with careful evaluation of the effect the initial magnetic moment has on the self-consistent solution of the electronic problem [79] , [80] . Adsorption energies are given relative to the M-N 4 defect with a total magnetic moment corresponding to the lowest electronic energy. M-N 4 , pyridinic N, and graphitic N sites were modeled using 4 × 4 orthorhombic single-layer graphene cell with the dimensions of 9.84 × 8.52 Å. Pyrrolic NH defect was modeled using a hexagonal single layer 17.04 × 17.04 Å unit cell. Structures of all the unit cells used for the DFT calculations are shown on Fig. S72 . A vacuum region of 20 Å was applied in all cases. All structures were optimized by allowing all atoms to relax (including adsorbents) while the cell parameters were kept fixed at the DFT optimized value for graphene. The criteria for the convergence of the electronic energy were set to 1 × 10 −5 eV. The forces were converged to 0.01 eV Å −1 . All calculations were performed as spin polarized calculations. The Pearson correlation coefficient was calculated using the python function np.corrcoef, which utilizes the equation below. R=∑(x_i-x̅) * (y_i-y̅)/√(∑(x_i-x̅)^2 * ∑(y_i-y̅)^2)
 Where R , is the correlation coefficient, x i and y i are the x and y values in samples, and \({\bar{x}}\) and \({\bar{y}}\) are mean values for the x and y variables. The computational approach for the calculation of Gibbs free energy of reactions and considered steps in the NO 3 RR and NO 2 RR mechanism are explained in details of our recent work [24] . However, it must be pointed out that all the Gibbs free energies were calculated at an experimentally determined pH of 6.3. We also emphasize that M-N-C catalysts are challenging to simulate, and the reliability of the computational results depends on many factors (e.g., see refs. [81] , [82] and SI note 4 ). Although one should pay attention to the accuracy of the absolute numbers, relative values and trends are more reliable.